Mechanical unzipping and rezipping of a single SNARE complex reveals hysteresis as a force-generating mechanism Formation of the soluble N-ethylmaleimide-sensitive factor attachment protein receptor (SNARE) complex provides mechanical thrust for membrane fusion, but its molecular mechanism is still unclear. Here using magnetic tweezers, we observe mechanical responses of a single neuronal SNARE complex under constant pulling force. Single SNARE complexes may be unzipped with 34 pN force. When rezipping is induced by lowering the force to 11 pN, only a partially assembled state results, with the C-terminal half of the SNARE complex remaining disassembled. Reassembly of the C-terminal half occurs only when the force is further lowered below 11 pN. Thus, mechanical hysteresis, characterized by the unzipping and rezipping cycle of a single SNARE complex, produces the partially assembled state. In this metastable state, unzipping toward the N-terminus is suppressed while zippering toward the C-terminus is initiated as a steep function of force. This ensures the directionality of SNARE-complex formation, making the SNARE complex a robust force-generating machine. SNARE (soluble N-ethylmaleimide-sensitive factor attachment protein receptor) proteins are thought to be the engine for intracellular membrane fusion in eukaryotic cells [1] , [2] , [3] , [4] , [5] . From a structural perspective, each SNARE protein carries one or two SNARE motifs, a heptad repeat composed of ~60 residues. Four SNARE motifs intertwine to form a parallel four-α-helix bundle called the SNARE complex. During synaptic vesicle fusion for neurotransmitter release, for example, synaptobrevin from the synaptic vesicle membrane forms a neuronal SNARE complex with syntaxin and SNAP-25 on the presynaptic membrane. SNARE-complex formation is suggested to proceed in sequential steps. The t-SNARE proteins, syntaxin and SNAP-25, form a binary precomplex first, which in turn serves as a scaffold for the binding of synaptobrevin [6] , [7] . As synaptobrevin is largely unstructured before binding to the t-SNARE precomplex [8] , [9] , [10] , [11] , [12] , SNARE complex formation can be essentially viewed as a protein folding process. The folding energy is large, which is used to bring two repelling membranes together to initiate fusion and to finally overcome the energy barriers for fusion pore opening. The SNARE complex is hence thought to be an inherent force-generating machine for membrane fusion. In this vein, the SNARE complex has been studied with several force spectroscopy techniques, including atomic force microscopy and surface force apparatus [13] , [14] , [15] , [16] , [17] . As tens of k B T (100–200 pN·nm) are estimated for the folding energy of the neuronal SNARE complex [14] , [18] , [19] , the force generated through the assembly of a single SNARE complex, with its contour length of 10 nm, should be in the order of tens of pN or even less. The large spring constant of atomic force microscopy, however, does not allow precise measurements at force levels below 100 pN. Using atomic force microscopy, a force of a few hundred pN was observed as the rupture force of single neuronal SNARE complexes, in which the SNARE complexes were pulled with a high loading rate of ~nN s −1 ( [13] , [15] , [17] ), which corresponds to a deeply non-equilibrium regime [20] . The surface force apparatus technique has produced important insights into the mechanics of SNARE proteins [14] , [16] . This technique, however, measured the force acting between two 10-μm 2 surfaces with >10 5 SNARE proteins involved in the surface–surface interaction. The mechanical characteristics of a single SNARE complex were then deduced by assuming models for the status of the SNAREs on the surface. However, the magnetic tweezers technique allows us to directly monitor the extension of a single molecule with nm accuracy [21] , [22] , [23] . Moreover, the force applied to each single molecule can be precisely controlled from sub-pN to tens of pN, which is robustly determined by the distance of the magnet from the sample [24] , [25] , [26] . Consequently, we were able to dissect the dynamic behaviour of a single neuronal SNARE complex while a well-calibrated, constant force was applied to the SNARE complex. The mechanical behaviour of a single SNARE complex showed a delicate dependence on different force levels and most importantly, substantial hysteresis in its assembly and disassembly, which we suggest makes the SNARE complex a force-generating machine with robust one-way zippering. Magnetic tweezers studying a single neuronal SNARE complex To probe the mechanical response of a single SNARE complex, we constructed a SNARE-DNA hybrid, in which 510 base-pair double-stranded DNAs were attached to the C-terminal ends (right after the +7 layer) of syntaxin 1 A and synaptobrevin 2 using a thiol-disulphide exchange reaction [27] , [28] , [29] ( Fig. 1a and Supplementary Fig. S2 ). Specifically, the DNA handles were attached to the exterior surface of the SNARE complex to minimize any perturbation to the formation of the four-helix bundle. We removed the Habc domain of syntaxin 1A and the transmembrane domains, but the entire SNARE motifs and linker regions of syntaxin 1A (amino acids 191–266) and synaptobrevin 2 (1–94) were included in our experiments (Methods and Supplementary Fig. S3 ). The −7 layer near the N-terminal end of the SNARE complex was covalently knotted by a cysteine-bridge for repetitive unzipping and rezipping experiments for a single molecule [28] ( Fig. 1b ). As the formation of the SNARE complex is thought to initiate in the N-terminal region and propagate toward the C-terminal ends, our positions for the DNA handles and cysteine-bridge knotting were chosen to induce unzipping in the C- to N-terminal direction and rezipping of a single SNARE complex in the opposite, N-to C-terminal direction. Thus, this rezipping process is designed to closely mimic the native zippering direction of the SNARE complex. This SNARE-DNA hybrid was connected to a polyethylene glycol-coated cover glass and a magnetic bead through biotin-neutravidin and dig-antidig linkages, respectively. 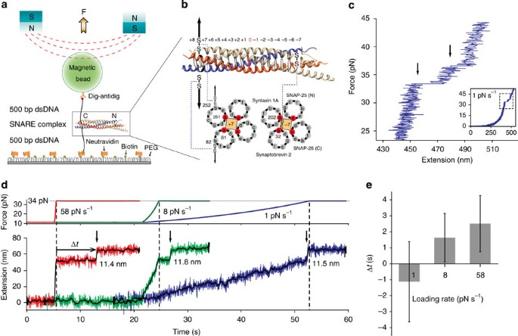Figure 1: Magnetic tweezers for studying the mechanical behaviour of a single neuronal SNARE complex. (a) Experimental scheme. The pulling force is generated by bringing a pair of magnets near a magnetic bead and is delivered to a single SNARE complex through DNA handles. The neuronal SNARE complex is composed of synaptobrevin 2 (blue coil), syntaxin 1A (red coil) and SNAP-25 (light yellow coils). (b) Detailed structure of the SNARE-DNA hybrid. The layered structure of the SNARE complex and the positions of the DNA handles and the internal disulphide bond are shown. The wheel diagrams of the +7 and −7 layers are shown, with the positions of the heptad repeats indicated by letters fromatog. (c) Representative force-extension trace of a single SNARE complex. An average loading rate of 1 pN s−1was used. The trace shows two sequential unzipping events (black arrows), and the inset shows the whole trace covering the force range from 0 to 50 pN. (d) Preliminary force-jump experiments. The pulling force was increased from 11–34 pN with three different loading rates of 1, 8 and 58 pN s−1, and was subsequently maintained at a constant force of 34 pN. The dashed line indicates the time when the force reaches 34 pN, and the arrow indicates unzipping events. The time lapse (Δt) was measured from the dashed line to the arrow in an individual trace. (e) Average Δtas a function of loading rate. The numbers of events (N) are 18, 15 and 119, and the numbers of SNARE complexes used (n) are 12, 7 and 41 for 1, 8 and 58 pN s−1, respectively. dsDNA, double-stranded DNA. Figure 1: Magnetic tweezers for studying the mechanical behaviour of a single neuronal SNARE complex. ( a ) Experimental scheme. The pulling force is generated by bringing a pair of magnets near a magnetic bead and is delivered to a single SNARE complex through DNA handles. The neuronal SNARE complex is composed of synaptobrevin 2 (blue coil), syntaxin 1A (red coil) and SNAP-25 (light yellow coils). ( b ) Detailed structure of the SNARE-DNA hybrid. The layered structure of the SNARE complex and the positions of the DNA handles and the internal disulphide bond are shown. The wheel diagrams of the +7 and −7 layers are shown, with the positions of the heptad repeats indicated by letters from a to g . ( c ) Representative force-extension trace of a single SNARE complex. An average loading rate of 1 pN s −1 was used. The trace shows two sequential unzipping events (black arrows), and the inset shows the whole trace covering the force range from 0 to 50 pN. ( d ) Preliminary force-jump experiments. The pulling force was increased from 11–34 pN with three different loading rates of 1, 8 and 58 pN s −1 , and was subsequently maintained at a constant force of 34 pN. The dashed line indicates the time when the force reaches 34 pN, and the arrow indicates unzipping events. The time lapse (Δ t ) was measured from the dashed line to the arrow in an individual trace. ( e ) Average Δ t as a function of loading rate. The numbers of events ( N ) are 18, 15 and 119, and the numbers of SNARE complexes used ( n ) are 12, 7 and 41 for 1, 8 and 58 pN s −1 , respectively. dsDNA, double-stranded DNA. Full size image An increasing level of force was applied to the SNARE-DNA hybrid by bringing a pair of magnets towards the magnetic bead ( Fig. 1a and Supplementary Fig. S1 ). While pulling the magnetic bead, we first monitored the extension of the SNARE-DNA hybrid as a function of the applied force. The SNARE-DNA hybrid extended smoothly until abrupt stepwise extensions were observed around 34 pN. As we had previously confirmed that the double-stranded DNA handles can be stretched smoothly without any stepwise changes up to ~65 pN (ref. 30 ), these stepwise changes in extension should indicate unzipping events of the single SNARE complex. For example, Fig. 1c shows a force-extension curve with two sequential unzipping steps near 35 pN while the force is increased from 0 to 50 pN with an average loading rate of 1 pN s −1 . It is remarkable that during these unzipping events, the force applied to a single SNARE complex essentially remains constant. In our magnetic tweezers, the magnet must move towards the magnetic beads by 100–200 μm to increase the force by 1 pN ( Supplementary Methods and Supplementary Fig. S1 ). Thus, the increases in SNARE extension by only about 10 nm due to the unzipping events do not essentially change the magnetic force experienced by the magnetic beads. This fact enables us to induce the unzipping and rezipping of a single SNARE complex at a constant pulling force without resorting to complicated feedback instruments, which is a unique feature of the magnetic tweezers technique. Intermediates in the unzipping of single SNARE complexes In the synaptic vesicle fusion process, the formation of SNARE complexes would proceed under defined levels of repulsion force between two fusing membranes. To gain insight into how a single SNARE complex behaves under such conditions, we first unzipped single SNARE complexes by applying a constant unzipping force of 34 pN (refs. 31 , 32 , 33 , 34 , 35 ). The force was increased from 11 pN, below which unzipping events were hardly ever observed ( Fig. 1c ), with three different loading rates of 1, 8 and 58 pN s −1 ( Fig. 1d ). In each pulling experiment, we measured the time lapse (Δ t ) from the moment that the force level reached 34 pN (dashed lines in Fig. 1d ) to the first unzipping event (arrows in Fig. 1d ). At a loading rate of 1 pN s −1 , Δ t has a slightly negative average of −1 s ( Fig. 1e ), reconfirming the unzipping force at 34 pN ( Supplementary Fig. S4 for the distribution of unzipping forces). We note that the sign of the average Δ t changes between the loading rate of 1 and 8 pN s −1 ( Fig. 1e ). This result indicates that with a loading rate larger than 8 pN s −1 , it is very likely that unzipping events in the SNARE-DNA hybrid will occur after the force level is set to 34 pN ( [36] ). Thus, if we use an even higher loading rate of 58 pN s −1 , there should be no hidden unzipping events during the force-jump to 34 pN. The first detected unzipping event consequently begins from the DNA anchor position at the C-terminal, +7 layer of the SNARE complex. By measuring the extensions due to unzipping, we can estimate the position in the SNARE complex at which the unzipping process has stopped. With the force-jump to 34 pN, we observed three types of unzipping events: one-step unzipping with a step size of ~10 nm ( Fig. 2a ), one-step unzipping with a larger step size of ~20 nm ( Fig. 2b ) and sequential two-step unzipping with two-step sizes of ~10 nm each ( Fig. 2c ) ( Supplementary Fig. S5 for more traces and Supplementary Fig. S6 for how we determine the step sizes). When we determined the step sizes of the first unzipping events regardless of whether there were second unzipping events or not, the resultant distribution showed two clear Gaussian distributions with peaks at 10.2 and 19.4 nm ( Fig. 2d ). In addition, when the first and second steps were summed for the two-step unzipping events, the distribution of this sum showed a single Gaussian distribution with a peak at 21.2 nm ( Fig. 2e ). 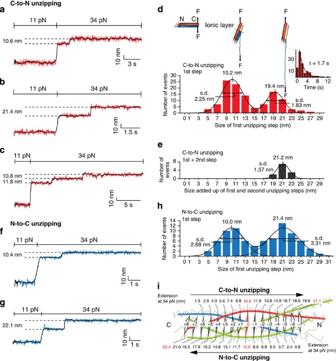Figure 2: Intermediates in the mechanical unzipping of a single SNARE complex. (a–c) Real-time traces showing C-to-N unzipping events of single SNARE complexes. The force was increased from 11 pN to 34 pN with loading rate of 58 pN s−1. The traces show one-step (a,b) or two-step unzipping events (c). (d) Distribution of the first unzipping steps of C-to-N unzipping experiment. Two Gaussian peaks were found at 10.2±0.1 nm (s.e.m.) and 19.4±0.2 nm (s.e.m.) (N=119 events fromn=41 SNARE complexes). The s.d. values are 2.25 and 1.83 nm, respectively. The distribution of the time lapse (Δt) was fitted using a single exponential equation with a decay time of 1.7 s (right inset). The anticipated structures of the SNARE complex are also shown. The cylinders represent the α-helical structure and the lines represent unstructured regions (blue: synaptobrevin 2, red: syntaxin 1A, light yellow: SNAP-25). (e) The sum of the first and second steps from the two-step unzipping events. The distribution shows one Gaussian peak at 21.2±0.01 nm (s.e.m.) with a s.d. of 1.37 nm (N=12 events fromn=7 SNARE complexes). (f,g) Real-time traces showing N-to-C unzipping events of single SNARE complexes. The force was increased from 11 to 34 pN with loading rate of 58 pN s−1. The traces show one-step unzipping with a size of ~10 nm (f) or ~20 nm (g). (h) Distribution of the first unzipping steps of N-to-C unzipping experiment. The distribution shows two Gaussian peaks at 10.0±0.2 nm (s.e.m.) and 21.4±0.2 nm (s.e.m.) (N=84 events fromn=25 SNARE complexes). The s.d. values are 2.68 nm and 3.31 nm, respectively. (i) Estimated extensions of a single SNARE complex when it is unzipped up to the specific layers from the respective DNA anchor positions. The extension values expected for C-to-N unzipping experiment are shown in the upper row, and the extensions for N-to-C unzipping experiment are shown in the bottom row. The extension values for the zeroth layer (ionic layer) and the knotted layers are shown in red. Figure 2: Intermediates in the mechanical unzipping of a single SNARE complex. ( a–c ) Real-time traces showing C-to-N unzipping events of single SNARE complexes. The force was increased from 11 pN to 34 pN with loading rate of 58 pN s −1 . The traces show one-step ( a , b ) or two-step unzipping events ( c ). ( d ) Distribution of the first unzipping steps of C-to-N unzipping experiment. Two Gaussian peaks were found at 10.2±0.1 nm (s.e.m.) and 19.4±0.2 nm (s.e.m.) ( N =119 events from n =41 SNARE complexes). The s.d. values are 2.25 and 1.83 nm, respectively. The distribution of the time lapse (Δ t ) was fitted using a single exponential equation with a decay time of 1.7 s (right inset). The anticipated structures of the SNARE complex are also shown. The cylinders represent the α-helical structure and the lines represent unstructured regions (blue: synaptobrevin 2, red: syntaxin 1A, light yellow: SNAP-25). ( e ) The sum of the first and second steps from the two-step unzipping events. The distribution shows one Gaussian peak at 21.2±0.01 nm (s.e.m.) with a s.d. of 1.37 nm ( N =12 events from n =7 SNARE complexes). ( f , g ) Real-time traces showing N-to-C unzipping events of single SNARE complexes. The force was increased from 11 to 34 pN with loading rate of 58 pN s −1 . The traces show one-step unzipping with a size of ~10 nm ( f ) or ~20 nm ( g ). ( h ) Distribution of the first unzipping steps of N-to-C unzipping experiment. The distribution shows two Gaussian peaks at 10.0±0.2 nm (s.e.m.) and 21.4±0.2 nm (s.e.m.) ( N =84 events from n =25 SNARE complexes). The s.d. values are 2.68 nm and 3.31 nm, respectively. ( i ) Estimated extensions of a single SNARE complex when it is unzipped up to the specific layers from the respective DNA anchor positions. The extension values expected for C-to-N unzipping experiment are shown in the upper row, and the extensions for N-to-C unzipping experiment are shown in the bottom row. The extension values for the zeroth layer (ionic layer) and the knotted layers are shown in red. Full size image To understand the structures of the SNARE complex represented by these peaks, the extension values were analysed using the worm-like chain model [28] , [29] ( Supplementary Methods and Supplementary Tables S1–S4 ). We assumed that under a high tension of 34 pN, synaptobrevin would lose its α-helicity when dissociated from the SNARE complex because synaptobrevin is thought to be mostly unstructured in its solitary form [8] , [9] , [10] , [11] , [12] . However, it is a wholly open question whether the t-SNARE precomplex and its putative α-helical structure are maintained even after the dissociation of synaptobrevin. To shed light on this question, we performed the same unzipping experiment in the reverse direction, in the N-to C-terminal direction. We chose the positions of the DNA handles and the disulphide bond to produce an extension very similar to the extension in the previous C-to-N unzipping experiment ( Supplementary Fig. S7 ). Remarkably, the N-to-C unzipping process also showed two Gaussian peaks for the step size of the first unzipping events ( Fig. 2f–h ). The higher peak is at 21.4 nm, a value very close to the 19.4-nm peak in Fig. 2d and the 21.2-nm peak in Fig. 2e . Our model estimates that the extensions of such fully unzipped SNARE complexes should have very different values, depending on the existence of the α-helical structure in the t-SNARE precomplex. An extension of ~20 nm is estimated when the precomplex structure is preserved, whereas ~30 nm is predicted when the α-helical precomplex becomes disassembled and syntaxin is further stretched ( Supplementary Tables S1–S4 ). As the higher peaks obtained from both C-to-N and N-to-C unzipping experiments consistently show extensions of ~20 nm, we assume that the precomplex structure is largely maintained even after the extraction of synaptobrevin by the 34-pN force. However, we cannot rule out an alternative model for the interpretation of our unzipping data. We further note that the positions of the lower Gaussian peaks also coincide, at 10.2 nm for C-to-N unzipping and 10.0 nm for N-to-C unzipping ( Fig. 2d ). With the assumptions made above for our model, these peaks at 10 nm exactly correspond to the partial unzipping up to the zeroth ionic layer ( Fig. 2i ). These partial-unzipping steps, however, show broad distributions around the 10-nm peaks, with s.d. values of 2.25 and 2.68 nm that correspond to the middle layers from the −2 to +2 layers ( Fig. 2d ). This result implies that each mechanical unzipping process stops at different positions, distributed through the middle layers between the −2 and +2 layers. Together, our observations support the hypothesis that the molecular interactions in these middle layers make a shared but important contribution to the stability of a single neuronal SNARE complex. 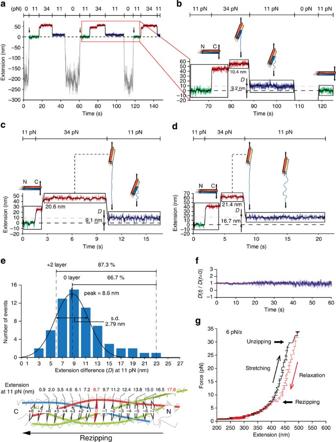Figure 3: Mechanical hysteresis produces the partially assembled state of a single SNARE complex. (a–d) Unzipping and rezipping cycles of a single SNARE complex. A fully assembled SNARE complex at 11 pN (green traces) was unzipped by the application of a 34-pN force (red traces). When the force was lowered back to 11 pN (blue traces), the extension was higher than the corresponding extension observed before the 34-pN unzipping. This extension difference (D) disappeared when the force was removed (0 pN) and then restored to 11 pN (next green traces). The upper insets are the anticipated structures of the SNARE complex. The cylinders represent the α-helical structure, and the lines represent the unstructured regions (blue: synaptobrevin 2, red: syntaxin 1A, light yellow: SNAP-25). (e) Distribution of the extension differences (D) with a Gaussian peak at 8.6±0.16 nm (s.e.m.) (N=63 force cycles fromn=33 SNARE complexes). The s.d. is 2.79 nm. The percentages of the rezipping processes that stalled before the ionic layer or before the +2 layer were 66.7% and 87.3%, respectively. At the bottom, the estimated extensions of a single SNARE complex under an 11-pN force are shown. (f) Time behaviour of the extension differences normalized by their initial values, that is,D(t)/D(t=0), wheretis the time spent in the second 11-pN phase (N=63 force cycles). In the statistical analyses ofeandf, we included only data for SNARE complexes that showed repetitive unzipping and rezipping events. (g) A representative force-extension trace of a single SNARE complex shows unzipping above 30 pN and rezipping below 10 pN (average loading rate of 6 pN s−1used). Mechanical hysteresis stabilizes partially assembled state Figure 3 illustrates the full cycles of our constant-force application experiments. By applying the unzipping force of 34 pN, we first unzipped a fully assembled SNARE complex as in the experiments illustrated in Fig. 2 ( Fig. 3a–d , red traces) and subsequently decreased the force back to 11 pN (blue traces) (hereafter, we use only the SNARE-DNA hybrid shown in Fig. 1 that shows C-to-N unzipping). Of note, the extension during this second 11-pN phase was higher than the extension during the first 11-pN phase before unzipping ( Fig. 3a–d , blue versus green traces; see Supplementary Fig. S8 for more traces), suggesting that parts of the SNARE motifs remained disassembled. When we completely removed the tension (0-pN force), the extension was restored to the original value of the fully assembled SNARE complex, indicating complete rezipping of the SNARE complex. The SNARE-DNA hybrid system was then ready for another cycle of the experiment ( Fig. 3a , arrows). Figure 3: Mechanical hysteresis produces the partially assembled state of a single SNARE complex. ( a–d ) Unzipping and rezipping cycles of a single SNARE complex. A fully assembled SNARE complex at 11 pN (green traces) was unzipped by the application of a 34-pN force (red traces). When the force was lowered back to 11 pN (blue traces), the extension was higher than the corresponding extension observed before the 34-pN unzipping. This extension difference ( D ) disappeared when the force was removed (0 pN) and then restored to 11 pN (next green traces). The upper insets are the anticipated structures of the SNARE complex. The cylinders represent the α-helical structure, and the lines represent the unstructured regions (blue: synaptobrevin 2, red: syntaxin 1A, light yellow: SNAP-25). ( e ) Distribution of the extension differences ( D ) with a Gaussian peak at 8.6±0.16 nm (s.e.m.) ( N =63 force cycles from n =33 SNARE complexes). The s.d. is 2.79 nm. The percentages of the rezipping processes that stalled before the ionic layer or before the +2 layer were 66.7% and 87.3%, respectively. At the bottom, the estimated extensions of a single SNARE complex under an 11-pN force are shown. ( f ) Time behaviour of the extension differences normalized by their initial values, that is, D ( t )/ D ( t =0), where t is the time spent in the second 11-pN phase ( N =63 force cycles). In the statistical analyses of e and f , we included only data for SNARE complexes that showed repetitive unzipping and rezipping events. ( g ) A representative force-extension trace of a single SNARE complex shows unzipping above 30 pN and rezipping below 10 pN (average loading rate of 6 pN s −1 used). Full size image We focused on the difference between the extensions at 11 pN observed before ( Fig. 3a–d , green traces) and after the 34-pN unzipping event (blue traces). This difference in extension ( D ) forms a rather broad distribution with one peak at 8.6 nm ( Fig. 3e ). However, there is no population at D =0, indicating that every rezipping process under the 11-pN force stops somewhere before reaching the DNA anchor position. Of particular note is the finding that the peak at 8.6 nm corresponds to the estimated extension of the C-terminal half of the SNARE complex, spanning from the DNA anchor position to the ionic layer, under the 11-pN force ( Fig. 3e and Supplementary Table S5 ). The percentages of the rezipping processes that stalled before the ionic layer or before the +2 layer were 66.7% and 87.3%, respectively, meaning that the remaining C-terminal parts would be left uncomplexed with the same probabilities ( Fig. 3e ). Moreover, 14% of the rezipping processes remained in the fully unzipped state ( D >15 nm) ( Fig. 3e and Supplementary Fig. S9 ). To test the stability of this extension difference, we normalized the extension differences of 63 force cycles by their initial values, that is, D ( t )/ D ( t =0) where t is the time spent in the second 11-pN phase. The average of these normalized extension differences was essentially maintained at unity within our observation time of 60 s ( Fig. 3f ). These observations suggest that at least the C-terminal half or even a larger part of the SNARE complex remains unzipped during the second 11-pN phase after the 34-pN unzipping ( Fig. 3a–d , blue traces). Our results clearly show that there is mechanical hysteresis in the unzipping and rezipping cycle of a single SNARE complex. We have demonstrated that the unzipping force of a single neuronal SNARE complex is ~34 pN. The 11-pN force is thus never large enough to unzip an assembled SNARE complex, but the same force of 11 pN is sufficient to prevent, in particular, the assembly of the C-terminal half of the SNARE complex. Indeed, when we obtained the force-extension curve while relaxing the force to 0 pN, the rezipping event was observed below 10 pN, which is smaller than the unzipping force by more than 20 pN ( Fig. 3g ). Using this large mechanical hysteresis, we were able to create the long-anticipated partially assembled state of a single neuronal SNARE complex, in which the N-terminal part was assembled while the C-terminal part remained disassembled. This partially assembled state is observed during the rezipping process in the N- to C-terminal direction, which mimics the native zippering of SNARE complexes. Finally, when the force was lowered by only a few pN from this stably-clamping 11-pN force, we observed the assembly of the C-terminal parts to complete the SNARE complex structure ( Fig. 4 ). To quantitatively characterize the SNARE-complex assembly from the partially assembled state, we repeated the force cycle experiment shown in Fig. 3 , but decreased the initial and final force levels from the original 11 pN to 9.1, 7.5 and 5.2 pN ( Fig. 4a–d ). The assembly of the C-terminal part was detected by a decrease in the extension, as confirmed by the restoration of the original extension of the fully assembled SNARE complex ( Fig. 4c , change from blue to green traces). 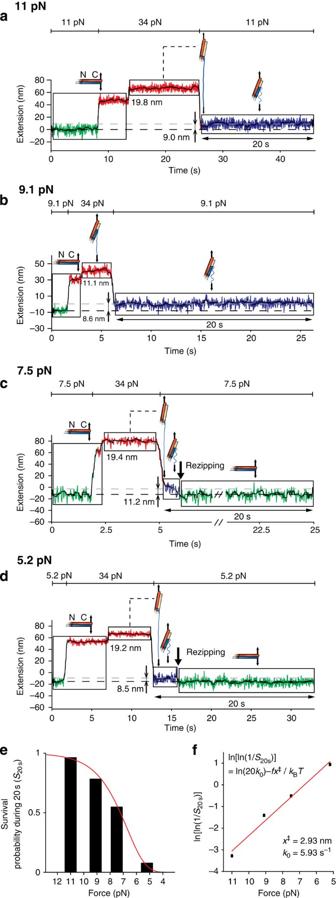Figure 4: Zippering of the C-terminal half of a single SNARE complex. (a–d) Force-cycle experiments for studying the C-terminal-half zippering of single SNARE complexes. By unzipping a single SNARE complex at 34 pN and subsequently lowering the force to 11 pN (a), 9.1 pN (b), 7.5 pN (c) and 5.2 pN (d), the SNARE complex can be trapped in its partially assembled state (blue traces). Then, during the observation time of 20 s, the extension difference is monitored to observe the occurrences of the C-terminal-half zippering, as indicated by the restoration of the original extension (changes from blue to green traces incandd). The fraction of partially assembled states that do not show such C-terminal zipping within the observation time is defined as the survival probability. (e) Survival probability after 20 s of observation () as a function of pulling force (N=27, 23, 31 and 26 events fromn=15, 11, 10 and 11 SNARE complexes for 11, 9.1, 7.5 and 5.2 pN, respectively). (f) Fitting the force dependence of the survival probability with equation (1) gives=2.93 nm and=5.93 s−1, whereis the position of the energy barrier confining the partially assembled state andis the kinetic rate for zippering of the C-terminal half at zero force. Figure 4: Zippering of the C-terminal half of a single SNARE complex. ( a – d ) Force-cycle experiments for studying the C-terminal-half zippering of single SNARE complexes. By unzipping a single SNARE complex at 34 pN and subsequently lowering the force to 11 pN ( a ), 9.1 pN ( b ), 7.5 pN ( c ) and 5.2 pN ( d ), the SNARE complex can be trapped in its partially assembled state (blue traces). Then, during the observation time of 20 s, the extension difference is monitored to observe the occurrences of the C-terminal-half zippering, as indicated by the restoration of the original extension (changes from blue to green traces in c and d ). The fraction of partially assembled states that do not show such C-terminal zipping within the observation time is defined as the survival probability. ( e ) Survival probability after 20 s of observation ( ) as a function of pulling force ( N =27, 23, 31 and 26 events from n =15, 11, 10 and 11 SNARE complexes for 11, 9.1, 7.5 and 5.2 pN, respectively). ( f ) Fitting the force dependence of the survival probability with equation (1) gives =2.93 nm and =5.93 s −1 , where is the position of the energy barrier confining the partially assembled state and is the kinetic rate for zippering of the C-terminal half at zero force. Full size image At each force level, we measured the survival probability of the partially assembled state during our observation time of 20 s ( ). This survival probability steeply diminished with decreasing force levels, indicating that the zippering process of the C-terminal part can be efficiently triggered by decreasing the pulling force below 11 pN ( Fig. 4e ). This force dependence of was well fitted to the equation ( Figure 4f and Supplementary Methods ). This fit gave =2.93 nm, the position of the energy barrier confining the partially assembled state, and =5.93 s −1 , which is the kinetic rate for zippering of the C-terminal part at zero force. Our results collectively suggest that the process of synaptic vesicle fusion is a delicate function of the repulsion force between the two fusing membranes ( Fig. 5 ). In the initial phase of membrane fusion, the two membranes are far apart, and the repulsion force on a single SNARE complex should be negligible ( Fig. 5a ). Our mechanical unzipping of single SNARE complexes reveals that the middle layers around the ionic layer are important for the mechanical stability of an individual SNARE complex. This result is consistent with the fact that the sequence of these middle layers, between the −2 and +2 layers, faithfully follows the leucine zipper model [37] , [38] . A fusion process would practically commence when those centre layers assemble to form a minimal, stable SNARE complex. With this SNARE complex formation, the repulsion force should steeply increase as the two fusing membranes are brought to nm-scale apposition. Most importantly, our results collectively suggest that if the effective repulsion force on a single SNARE complex becomes larger than 11 pN (but smaller than 34 pN), each SNARE complex will be trapped in the ‘partially assembled’ state without requiring any help from other auxiliary proteins ( Fig. 5b ). 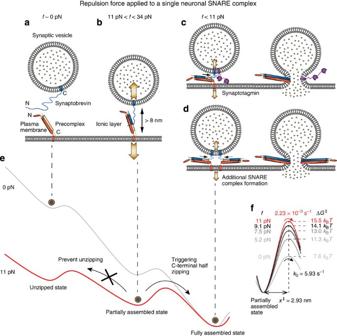Figure 5: Model for synaptic vesicle fusion based on our mechanical study of single SNARE complexes. (a–d) Model for synaptic vesicle fusion. In the initial phase of synaptic vesicle fusion, the two membranes are far apart and the repulsion force on a single SNARE complex should be negligible (a). When the effective repulsion on a single SNARE complex is larger than 11 pN (but smaller than 34 pN), the SNARE complex becomes trapped in the partially assembled state, in which the C-terminal half of the SNARE motif is selectively disassembled (b). Zippering of the remaining C-terminal half can be triggered by the work of fusion regulators such as synaptotagmin (c) and/or the formation of additional SNARE complexes (d). (e) Energy landscape diagrams for the SNARE-complex formation at 0-pN and 11-pN forces. (f) Energy barriers separating the partially assembled state from the fully assembled state of a single SNARE complex. The parameters of the energy barrier,,and, are shown for various force values. Figure 5: Model for synaptic vesicle fusion based on our mechanical study of single SNARE complexes. ( a – d ) Model for synaptic vesicle fusion. In the initial phase of synaptic vesicle fusion, the two membranes are far apart and the repulsion force on a single SNARE complex should be negligible ( a ). When the effective repulsion on a single SNARE complex is larger than 11 pN (but smaller than 34 pN), the SNARE complex becomes trapped in the partially assembled state, in which the C-terminal half of the SNARE motif is selectively disassembled ( b ). Zippering of the remaining C-terminal half can be triggered by the work of fusion regulators such as synaptotagmin ( c ) and/or the formation of additional SNARE complexes ( d ). ( e ) Energy landscape diagrams for the SNARE-complex formation at 0-pN and 11-pN forces. ( f ) Energy barriers separating the partially assembled state from the fully assembled state of a single SNARE complex. The parameters of the energy barrier, , and , are shown for various force values. Full size image We note that while our manuscript was under review, a similar report on the mechanical behaviour of single SNARE complexes was published [39] . In that work based on the optical tweezers technique, the partially assembled state was also observed as an intermediate during the unzipping processes. Another unzipping intermediate was resolved, in which the linker regions were unzipped before unzipping of the C-terminal half of the SNARE motifs [39] . After full unzipping, the SNARE complexes were subsequently relaxed by gradually lowering the tension. In contrast to the unzipping process with multiple intermediates, the rezipping process occurred in one-step without showing any intermediates. In our work, however, we observed the partially assembled state in the course of the rezipping process. This observation has been made possible by force-jump experiments, a unique experimental design using the magnetic tweezers technique because it has an effective stiffness (~10 −2 pN μm −1 ) far smaller than that of the optical tweezers and thus readily allows for constant force application [24] , [25] , [26] , [40] . We demonstrate for the first time that despite its huge folding energy, the zippering process of a single SNARE complex can be stalled at the partially assembled state over a wide force range between 11 pN and 34 pN. While the previous report using optical tweezers provides ultra-structural details of the unzipping process, our work reports on the mechanical behaviour of a single SNARE complex during rezipping in unprecedented details. This partially assembled intermediate could be an ideal state of the primed synaptic vesicles because, upon Ca 2+ influx, only the zippering of the remaining C-terminal half is needed to complete the fusion. This minimal requirement for protein actions, a folding transition in already-bound protein complexes, may essentially allow for a millisecond-scale response of neurotransmitter release. In such a partially assembled state, our work shows that the distance between the transmembrane domains of syntaxin and synaptobrevin is at least larger than 8 nm ( Fig. 5b ). This information poses an intriguing question as to the corresponding structure of fusing membranes. One simple but plausible scenario is that, as recently observed, the two membranes may be separated or may make a minimal point contact [41] , [42] . Alternatively, the membranes may make an extensive contact in a hemifused state, and their contact area may be lined by multiple copies of partially assembled SNARE complexes that exert tension on one another. Either way, our force-titration data in Fig. 4 demonstrate that zippering of the C-terminal half can be triggered by lowering the tension by only a few pN from the 11-pN force. For example, when the tension was reduced from 11 to 5.2 pN, the kinetic rate for the C-terminal-half zippering was increased by more than two orders of magnitude. To mitigate the repulsion force, a fusion regulator would energetically attract both of the fusing membranes ( Fig. 5c ). Synaptotagmin is a prominent example, which has been reported to bridge two membranes with a high affinity in response to Ca 2+ ions [43] , [44] , [45] . The addition of newly formed SNARE complexes also distributes the tension and lowers the effective repulsion force applied to a single SNARE complex ( Fig. 5d ). We anticipate that the repulsion forces will be substantially different from system to system because different fusion systems have disparate lipid compositions, membrane curvatures, available accessory proteins and types of SNARE proteins involved in vesicle fusion. This possibility explains why many different numbers of SNARE complexes have been reported to be required for efficient fusion [46] , [47] , [48] , [49] , [50] . However, as long as the same SNARE complex constitutes the core engine for membrane fusion, the threshold triggering the assembly of the C-terminal half will always exist at the same force level, for example, at 11 pN in the case of the neuronal SNARE complex. We suggest that the mechanical behaviour of a single SNARE complex described in this work provides a more unified and fundamental viewpoint on different fusion processes than would be possible with the number of SNARE complexes. From the perspective of the folding landscape, the partially assembled state is a metastable intermediate induced by mechanical force [51] . At zero force, the entire folding landscape of the SNARE complex is steeply tilted toward the fully assembled state due to the deep folding energy of the SNARE complex ( Fig. 5e , 0-pN energy landscape). Our mechanical unzipping data suggest that the free energy of the unzipped state becomes lower than the free energy of the fully assembled state only when the high unzipping force of 34 pN is applied ( Supplementary Fig. S9 ). Thus, under the threshold force of 11 pN, which is more than 20 pN lower than the unzipping force, the overall landscape should still be strongly biased toward the fully assembled state ( Fig. 5e , 11-pN energy landscape). This situation effectively prevents a backward transition of the partially assembled state to the unzipped state, meaning that an unzipping process toward the N-terminus is very unlikely to occur from the partially assembled state. At the same time, an energy barrier separates the partially assembled state from the fully assembled state, which prevents zippering of the C-terminal half of the SNARE motifs. Our single-molecule force spectroscopy experiments determined that this energy barrier is 7.61 k B T at zero force, separated from the partially assembled state by a distance of 2.93 nm ( Fig. 5f ). Because of this large distance, the energy barrier is substantially fortified by a small change in force (the lever-arm effect), for example, up to 15.5 k B T at the 11-pN force. At the same time, the energy barrier quickly shrinks as the repulsion force is reduced. Consequently, the kinetic rate of the C-terminal-half zipping is estimated to be as low as 2.23 × 10 −3 s −1 at 11 pN, but increases to 5.93 s −1 at zero force, larger by a factor of more than three orders of magnitude. This result implies that when a force greater than 10 pN is applied, the lifetime of the partially assembled state is long enough to be observed. In traditional biochemistry approaches that are performed under essentially tension-free environments, the partially assembled state would be too short-lived to detect which may explain why the existence of the partially assembled state of the neuronal SNARE complex has previously been elusive. Finally, we note that the physical origin of this energy barrier needs to be understood. We speculate that it involves a cooperative formation of α-helix in the SNARE motif of synaptobrevin. The hysteresis in SNARE-complex assembly and disassembly has been observed by both thermal and chemical methods [52] . We demonstrate here a large hysteresis in the mechanical unzipping and rezipping of a single SNARE complex as a function of the pulling force. This mechanical hysteresis is of particular interest because SNARE proteins, as force-generating proteins, are naturally working under force-loaded environments. The large mechanical hysteresis permits the observation of the partially assembled state at a relatively low level of tension. In this metastable state, unzipping towards the N-terminus is strongly suppressed, while zippering toward the C-terminus is initiated as a steep function of the repulsion force. In other words, the partially assembled state has the effect of rectifying the direction of SNARE-complex formation, firmly pushing SNARE zippering towards the transmembrane domains at the C-terminal end. Protein expression and purification All SNARE proteins were expressed in the E. coli Rosetta (DE3) pLysS (Novagen) cell strain: syntaxin 1A (amino acids 191–266, SNARE motif with C-terminal linker), SNAP-25 (amino acids 1–206 with four native cysteines replaced by alanines) and synaptobrevin 2 (amino acids 1–94 lacking the transmembrane domain). Cells containing the glutathione S -transferase-tagged neuronal SNARE proteins were grown at 37 °C in LB medium with 100 μg ml −1 ampicillin until the absorbance at 600 nm (A600) reached 0.6–0.8. Isopropyl-β-D-thiogalactopyranoside was added to a final concentration of 0.5 mM, and the cells were further grown at 16 °C overnight. The cell pellets were collected by centrifugation at 6 000 g for 10 min and resuspended in 10 ml PBS (pH 7.4) containing 1% (w/v) N-lauroylsarcosine sodium salt, 2 mM 4-(2-aminoethyl) benzenesulfonyl fluoride hydrochloride and 5 mM dithiothreitol. The cells were lysed by sonication on ice and centrifuged at 15,000 g for 30 min at 4 °C. The cell lysate was mixed with 1 ml glutathione-agarose beads and nutated for 1 h at 4 °C. After binding, the beads were washed with PBS. The proteins were then cleaved with 30 U ml −1 thrombin for 1 h at room temperature and eluted from the beads with PBS. The purified proteins were analysed by 12% SDS–polyacrylamide gel electrophoresis ( Supplementary Fig. S2a ). Certain residues in the C-terminal ends of syntaxin 1A and synaptobrevin 2 (right after the +7 layer) were replaced with cysteines to attach DNAs by a thiol-disulphide exchange reaction [27] , [28] , [29] (amino acid 252 for syntaxin 1A and amino acid 82 for synaptobrevin 2, both corresponding to position b of the heptad repeat). As these residues in position b are on the exterior surface of the SNARE complex ( Fig. 1b ), we can attach the DNA handles while minimizing perturbation to the formation of the four-helix bundle. Selected residues in the −7 layer were also replaced with cysteines for the repetitive single-molecule unzipping and rezipping experiments (amino acid 202 for syntaxin 1A and amino acid 32 for synaptobrevin 2 in position a of the heptad repeat). As these residues in position a are in close contact with one another ( Fig. 1b ), the disulphide bond spontaneously formed to knot the N-terminal end of the SNARE complex [28] . For the N- to C-terminal unzipping experiments, amino acids 200 and 254 for syntaxin 1A and amino acids 30 and 84 for synaptobrevin 2 were replaced with cysteines ( Supplementary Fig. S7 ). SNARE-DNA hybrids To prepare the DNA handles, two types of 510-bp DNA handles were PCR-amplified to obtain large quantities (each, ~70 μg in 1.6 ml). For PCR amplification, λ DNA template, forward primers with a 5′-thiol group and reverse primers with either 5′-biotin or 5′-digoxigenin were used. The PCR products were activated with 10 mM 2,2′-dithiodipyridine (DTDP) for thiol-disulphide exchanges for 12 h at 37 °C and purified with PBS ( [27] , [28] , [29] ) Each handle was concentrated to ~10 μM using Amicon Ultra-0.5 centrifugal filters. The two types of DNA handles were mixed at an equal ratio, and the mixture was stored at 2 °C. To form SNARE complexes (42 kDa), a 1:1:1 mixture of syntaxin 1 A (amino acids 191–266, 9 kDa), SNAP-25 (23 kDa) and synaptobrevin 2 (amino acids 1–94, 10 kDa) was incubated with 10 mM dithiothreitol for 1 h at room temperature and purified with PBS using a PD MiniTrap G-25 desalting column (GE Healthcare). Domain-swapped SNARE complexes (> 84 kDa) were removed using Amicon Ultra-0.5 centrifugal filters (UFC505024). The SNARE complexes were reacted with 2,2′-dithiodipyridine-activated DNA handles for 3 h at room temperature, and the DNA handles were then covalently linked to the SNARE complexes to form the ‘SNARE-DNA hybrid’. The SNARE complexes and the SNARE-DNA hybrids were analysed, respectively, by 12% SDS–polyacrylamide gel electrophoresis and 1.3% Tris-acetate-EDTA (TAE) agarose gel ( Supplementary Fig. S2 ). Single-molecule force spectroscopy Single-molecule magnetic tweezers were built based on a home-made inverted microscope. The magnetic field is generated by a pair of permanent magnets located above the sample stage, and the force applied to the magnetic beads is controlled by the vertical position of the magnets ( Supplementary Fig. S1a ). The force was calibrated by analysing the lateral fluctuations of the magnetic beads, which were tethered to the surface by a 16.5-μm-long λ DNA tether ( Supplementary Fig. S1b ). To this end, the following equation was used: where is the thermal energy; is the extension of the DNA tether; and represents the lateral fluctuations of the bead [21] , [53] ( Supplementary Methods and Supplementary Fig. S1c ). The flow cell consisted of two sandwiched cover glasses fixed by double-sided tape. The bottom surface was coated with polyethylene glycol to prevent nonspecific binding of the proteins and beads [44] . The reagents were sequentially injected to the flow cell in the following order: neutravidin (Invitrogen), SNARE-DNA hybrid, 1-μm polystyrene beads coated with streptavidin (Polysciences) and 2.8-μm magnetic beads coated with anti-digoxigenin (Dynal M-270). The incubation took place at room temperature, and after each incubation step, the flow cell was washed with PBS buffer. A number of 1-μm polystyrene non-magnetic beads were immobilized directly on the bottom surface and used as references in correcting the lateral and vertical position of the magnetic beads. The magnetic beads were illuminated by a blue light-emitting diode. The diffraction patterns from the beads (concentric rings alternating in brightness) were image-captured at a 60-Hz frame rate by a CCD camera (JAI CM-040GE). We can track in real-time the lateral and vertical positions of the beads by observing the movement of the centre and the expansion (or shrinkage) of the diffraction patterns, respectively. This tracking was performed using custom-written tracking software [22] , [53] . From each acquired image, the lateral centre position ( x , y ), the vertical extension ( z ) and the radial averaged intensity profiles I ( r ) of the diffraction patterns were calculated and stored. In the diffraction method, the extension z was calculated from previously acquired calibration images. We selected a suitable SNARE-DNA hybrid sample by real-time monitoring of the force-extension curve and by observing the responses of the magnetic bead while approaching and rotating the magnet [54] . The step sizes of the unzipping and rezipping events were determined as the differences between the arithmetic mean values of the data. The error in our step-size measurement is smaller than 1 nm for both the unzipping and rezipping events ( Supplementary Methods and Supplementary Fig. S6 ). A median filter with 250–500-ms windows was applied to the extension traces to present the stepwise events more clearly. How to cite this article: Min, D. et al . Mechanical unzipping and rezipping of a single SNARE complex reveals hysteresis as a force-generating mechanism. Nat. Commun. 4:1705 doi: 10.1038/ncomms2692 (2013).